Capturing carbon dioxide as a polymer from natural gas Natural gas is considered the cleanest and recently the most abundant fossil fuel source, yet when it is extracted from wells, it often contains 10–20 mol% carbon dioxide (20–40 wt%), which is generally vented to the atmosphere. Efforts are underway to contain this carbon dioxide at the well-head using inexpensive and non-corrosive methods. Here we report nucleophilic porous carbons are synthesized from simple and inexpensive carbon–sulphur and carbon–nitrogen precursors. Infrared, Raman and 13 C nuclear magnetic resonance signatures substantiate carbon dioxide fixation by polymerization in the carbon channels to form poly(CO 2 ) under much lower pressures than previously required. This growing chemisorbed sulphur- or nitrogen-atom-initiated poly(CO 2 ) chain further displaces physisorbed hydrocarbon, providing a continuous carbon dioxide selectivity. Once returned to ambient conditions, the poly(CO 2 ) spontaneously depolymerizes, leading to a sorbent that can be easily regenerated without the thermal energy input that is required for traditional sorbents. An automobile operating on natural gas produces ~30% lower carbon dioxide (CO 2 ) emissions than when operating on gasoline [1] . Provided technological efficiencies are maintained to minimize direct natural gas leakage to the atmosphere, there is a significant lowering of greenhouse gas emissions when using natural gas rather than liquid hydrocarbons [2] , [3] . At the same time, natural gas wells have typical CO 2 concentrations of 10–20 mol%, and that can rise to as high as 70 mol% in some locations [3] . The CO 2 is generally vented into the atmosphere at natural gas collection stations, significantly offsetting the environmental advantages of using natural gas as a fuel. Typically, aqueous amine scrubbers are used to remove CO 2 from natural gas, but aqueous amines are corrosive, and the CO 2 -containing liquid requires heating to 125–140 °C to liberate the CO 2 from the amine carbonate. This heating demands a high energy input and the scrubbers are not easily amenable to offshore CO 2 capture due to their size and weight [4] , [5] . Long and other groups extensively reviewed aqueous amines and other methods of CO 2 capture that include metal oxide frameworks, zeolites, ionic liquids, cryogenic distillation, membranes and metal oxides [6] , [7] , [8] , [9] . Some of these have hydrolytic instabilities and/or low densities leading to low volumetric efficiencies, or sometimes poor selectivity relative to methane, but most often there are synthesis constraints or energy costs associated with these technologies that lessen their suitability for on-site CO 2 capture from natural gas. Here we report new materials from simple and inexpensive carbon–sulphur or carbon–nitrogen solid sorbents, which separate CO 2 from natural gas, with 0.82 g CO 2 per g of sorbent (82 wt%) captured at 30 bar. A mechanism is described where CO 2 is polymerized in the channels of the support, as initiated by the sulphur or nitrogen atoms that are part of the carbon framework. No temperature swing is needed; it proceeds at ambient temperature. Eventually, heat transfer between cylinders during the exothermic sorption and endothermic desorption might provide the requisite thermodynamic exchanges. The process uses the inherent natural gas-well pressure of 200–300 bar as a driving force during the polymerization. By lowering the pressure back to ambient conditions after CO 2 uptake, the poly(CO 2 ) then depolymerizes where it can be off-loaded, or pumped back downhole into the structures that had held it for geological timeframes. Synthesis and characterization of porous carbons Sulphur- and nitrogen-containing porous carbons (SPC and NPC, respectively) were prepared by treating bulk precursor polymers with potassium hydroxide (KOH) at 600 °C ( Fig. 1a ; refs 10 , 11 ). The resulting products were solid porous carbon materials with homogeneously distributed sulphur or nitrogen atoms incorporated into the carbon framework. They exhibited pores and channel structures as well as high surface areas of 2,500 and 1,490 m 2 g −1 (N 2 , Brunauer–Emmett–Teller) for the SPC and the NPC, respectively, with pore volumes of 1.01 cm 3 g −1 and 1.40 cm 3 g −1 , respectively. The scanning electron microscopy and transmission electron microscopy (TEM) images are shown in Fig. 1b–d , and the X-ray photoelectron spectroscopy (XPS) analyses are shown in Supplementary Fig. 1 . 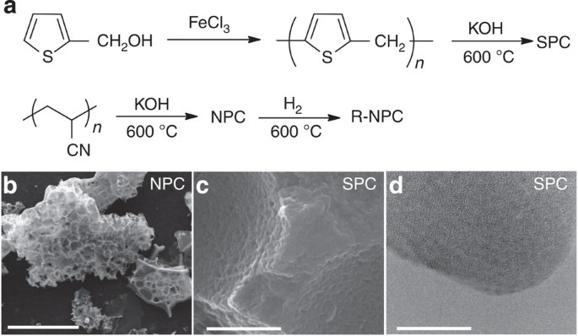Figure 1: The synthetic schemes and micrographic images. (a) The synthesis of SPC or NPC by treating poly[(2-hydroxymethyl)thiophene] or poly(acrylonitrile) with KOH at 600 °C and then washing with dilute HCl and water until the extracts are neutral. The NPC is further reduced using 10% H2at 600 °C to form R-NPC, see Methods. (b) Scanning electron microscopy (SEM) image of NPC. Scale bar, 100 μm. (c) SEM image of SPC. Scale bar, 500 nm. (d) TEM image of the SPC. Scale bar, 25 nm. Figure 1: The synthetic schemes and micrographic images. ( a ) The synthesis of SPC or NPC by treating poly[(2-hydroxymethyl)thiophene] or poly(acrylonitrile) with KOH at 600 °C and then washing with dilute HCl and water until the extracts are neutral. The NPC is further reduced using 10% H 2 at 600 °C to form R-NPC, see Methods. ( b ) Scanning electron microscopy (SEM) image of NPC. Scale bar, 100 μm. ( c ) SEM image of SPC. Scale bar, 500 nm. ( d ) TEM image of the SPC. Scale bar, 25 nm. Full size image CO 2 uptake measurements Although CO 2 has no liquid state at ambient conditions, it can easily liquefy when the system pressure is higher, which can cause a serious analytical error during the measurements [12] , [13] . Since there are presently no accepted standards for CO 2 uptake measurements [14] , further verification was sought: the same samples were analysed using different volumetric analysis instruments at Rice University and at the National Institute of Standards and Technology (NIST), and these were further confirmed with gravimetric measurements [15] . 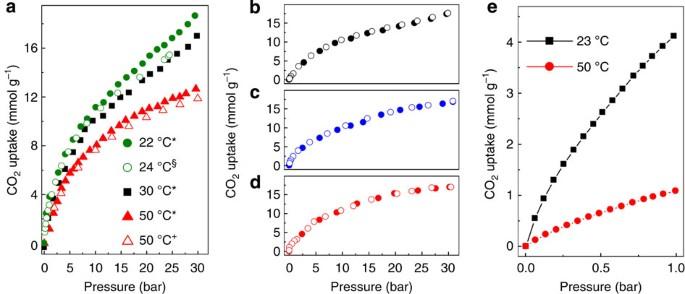Figure 2: CO2uptake measurements. (a) Volumetric and gravimetric uptake of CO2on SPC at different temperatures and pressures. Those designated with ‘*’ were recorded volumetrically at Rice University. That designated with ‘§’ was performed volumetrically at NIST. That designated ‘+’ was measured gravimetrically at NIST. All gravimetric measurements were corrected for buoyancy. (b–d) Three consecutive CO2sorption–desorption cycles on the SPC over a pressure range from 0 to 30 bar at 30 °C. All solid circles indicate CO2sorption, while the open circles designate the desorption process. (e) Volumetric SPC CO2sorption isotherms at 23 °C and 50 °C over a pressure range from 0 to 1 bar. Figure 2 shows the pressure-dependent CO 2 excess uptake for the SPC sorbent at different temperatures peaking at 18.6 mmol CO 2 per g of sorbent (82 wt%) when at 22 °C and 30 bar. The sorption results measured by volumetric and gravimetric analyses were comparable, as were those measurements on the two volumetric instruments. We chose 30 bar as the upper pressure limit in our experiments because a 300-bar well-head pressure at 10 mol% CO 2 concentration would have a CO 2 partial pressure of 30 bar. Figure 2b–d shows three consecutive CO 2 sorption–desorption cycles on SPC over a pressure range from 0 to 30 bar, which indicates that the SPC could be regenerated using a pressure swing process while retaining its original CO 2 sorption capacity. Figure 2: CO 2 uptake measurements. ( a ) Volumetric and gravimetric uptake of CO 2 on SPC at different temperatures and pressures. Those designated with ‘*’ were recorded volumetrically at Rice University. That designated with ‘§’ was performed volumetrically at NIST. That designated ‘+’ was measured gravimetrically at NIST. All gravimetric measurements were corrected for buoyancy. ( b – d ) Three consecutive CO 2 sorption–desorption cycles on the SPC over a pressure range from 0 to 30 bar at 30 °C. All solid circles indicate CO 2 sorption, while the open circles designate the desorption process. ( e ) Volumetric SPC CO 2 sorption isotherms at 23 °C and 50 °C over a pressure range from 0 to 1 bar. Full size image In the case of microporous materials with negligible external surface area, total uptake is often used as an approximation for absolute uptake, and the two values here are within 10% of each other; for example, the absolute CO 2 uptake of the SPC was 20.1 and 13.9 mmol g −1 under 30 bar at 22 °C and 50 °C, respectively ( Supplementary Figs 2 and 3 and Supplementary Note 1 ). Similarly, although absolute adsorption isotherms can be used to determine the heat of sorption, excess adsorption isotherms are more often used to calculate the heat of CO 2 sorption (Q CO2 ) before the critical point of the gas [16] , [17] . Thus, the excess CO 2 sorption isotherms measured at two different temperatures, 23 °C and 50 °C ( Fig. 2e ), were input into the Clausius–Clapeyron equation [18] (see Supplementary Note 2 ). At lower surface coverage (≤1 bar), which could be expected to be more indicative of the sorbate–sorbent interaction, the SPC exhibits a heat of CO 2 sorption of 57.8 kJ mol −1 . Likewise, the maximum Q CO2 values for nucleophile-free porous materials, such as activated carbon, Zeolite 5 A and zeolitic imidazolate framework (ZIF-8, a class of the metal oxide frameworks) were measured to be 28.4, 31.2 and 25.6 kJ mol −1 , respectively, at low surface coverage (see Supplementary Table 1 ). Based on this data, the SPC possesses the highest CO 2 sorption enthalpy among these complementary sorbents measured at low surface coverage. In order to better assess the sorption mechanism during the CO 2 uptake, attenuated total reflectance infrared spectroscopy (ATR-IR) was used to characterize the properties of the sorbents before and after the CO 2 uptake. A sample vial with ~100 mg of the SPC was loaded into a 0.8 l stainless steel autoclave equipped with a pressure gauge and valves. Before the autoclave was sealed, the chamber was flushed with CO 2 (99.99%) to remove residual air, and the system was pressurized to 10 bar (line pressure limitation). The sorbent was therefore isobarically exposed to CO 2 in the closed system at 23 °C. After 15 min, the system was vented to nitrogen at ambient pressure and the sorbent vial was immediately removed from the chamber and the sorbent underwent ATR-IR and Raman analyses in air. 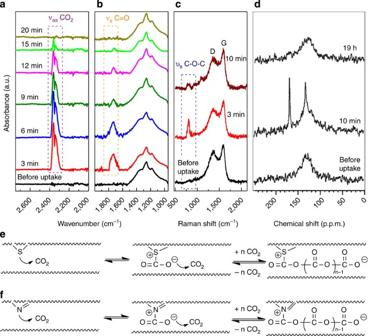Figure 3: Spectral changes before and after sorption–desorption and polymerization mechanism. (a,b) ATR-IR, (c) Raman and (d) 50.3 MHz13C MAS NMR spectra before and after CO2sorption at 10 bar and room temperature. All spectra were recorded at the elapsed times indicated on the graphs after the SPC sorbent was returned to ambient pressure. In the NMR experiments, the rotor containing the SPC was tightly capped during the analyses. For the 19 h NMR experiment the same material was left under ambient conditions for 19 h before being repacked in the rotor to obtain the final spectrum. Each NMR spectrum took 80 min to record. (e,f) A mechanism that illustrates the poly(CO2) formation in SPC or NPC, respectively, in a higher pressure CO2environment. With the assistance of the nucleophile, such as S or N, the CO2polymerization reaction is initiated under pressure, and the polymer is further likely stabilized by the van der Waals interactions with the carbon surfaces in the pores. Figure 3a,b shows the ATR-IR spectra of the SPC before (black line) and after exposure to 10 bar of CO 2 followed by ambient conditions for the indicated times. The two regions that appear in the ATR-IR spectra (outlined by the dashed-line boxes) after the CO 2 sorption are of interest. The first IR peak, located at 2,345 cm −1 , is assigned to the anti-symmetric CO 2 stretch, confirming that CO 2 was physisorbed and evolving from the SPC sorbent. The other IR band, centred at 1,730 cm −1 , is attributed to the C=O symmetric stretch from the poly(CO 2 ) on the SPC. Interestingly, this carbonyl peak is only observed with the porous heteroatom-doped carbon, such as the SPC and NPC. Other porous sorbents without nucleophilic species, such as ZIF-8 and activated carbon, only showed the physisorbed or evolving CO 2 peak (~2,345 cm −1 ) ( Supplementary Figs 4 and 5 ). Once the CO 2 -filled SPC returned to ambient pressure, the key IR peaks attenuated over time and disappeared after 20 min. Based on this data, the ATR-IR study confirmed the poly(CO 2 ) formation. Raman spectroscopy was further used to probe individual chemical bond vibrations as shown in Fig. 3c . The carbonaceous graphitic G-band and defect-derived diamondoid D-band were at 1,590 and 1,350 cm −1 (refs 19 , 20 ). The peak at 798 cm −1 can be attributed to the symmetric stretch of the C–O–C bonds [21] , [22] , which was not observed for the other nucleophile-free porous materials, suggesting that the poly(CO 2 ), with the –(O–C(=O)) n – moiety, was formed. The monothiocarbonate and carbamate anions within the channels of the SPC and NPC, respectively, were the likely initiation points for the CO 2 polymerization since no poly(CO 2 ) was seen in activated carbon ( Supplementary Fig. 5 ). Furthermore, 13 C NMR also confirms the presence of the poly(CO 2 ) formation. The sorbent gives a broad signal characteristic of aromatic carbon ( Fig. 3d , bottom). After exposure to CO 2 , a relatively sharp signal on top of the broad sorbent signal appears at 130.6 p.p.m., which can be assigned to the CO 2 that is evolving from the support. A sharp signal also appears at 166.5 p.p.m. ( Fig. 3d , middle), which is characteristic of the carbonyl resonance for poly(CO 2 ). Both of these signals are gone 19 h later ( Fig. 3d , top), see Supplementary Note 3 . Figure 3: Spectral changes before and after sorption–desorption and polymerization mechanism. ( a , b ) ATR-IR, ( c ) Raman and ( d ) 50.3 MHz 13 C MAS NMR spectra before and after CO 2 sorption at 10 bar and room temperature. All spectra were recorded at the elapsed times indicated on the graphs after the SPC sorbent was returned to ambient pressure. In the NMR experiments, the rotor containing the SPC was tightly capped during the analyses. For the 19 h NMR experiment the same material was left under ambient conditions for 19 h before being repacked in the rotor to obtain the final spectrum. Each NMR spectrum took 80 min to record. ( e , f ) A mechanism that illustrates the poly(CO 2 ) formation in SPC or NPC, respectively, in a higher pressure CO 2 environment. With the assistance of the nucleophile, such as S or N, the CO 2 polymerization reaction is initiated under pressure, and the polymer is further likely stabilized by the van der Waals interactions with the carbon surfaces in the pores. Full size image Compared with secondary amine-based CO 2 sorbents where maximum capture efficiency is 0.5 mol CO 2 per mol N (2 RNH 2 +CO 2 →RNH 3 + − O 2 CNHR), the SPC and NPC demonstrate a unique mechanism during the CO 2 uptake process resulting in their remarkably higher CO 2 capacities versus S or N content (8.1 atomic % of S and 6.2 atomic % of N in the SPC and NPC, respectively, by XPS analysis). Figure 3e,f shows a mechanism to illustrate this CO 2 fixation by polymerization. Dimeric CO 2 uptake has been crystallographically observed in metal complexes [22] , and polymeric CO 2 has been detected previously but only at extremely high pressures of ~15,000 bar (ref. 21 ). The spectroscopic determination here confirms poly(CO 2 ) formation at much lower pressures than formerly observed. A series of porous materials with and without the nucleophilic heteroatoms were tested to compare their CO 2 capture performance up to 30 bar at 30 °C ( Fig. 4a ). The SPC had the highest CO 2 capacity; the NPC, activated carbon, zeolite 5A and ZIF-8 had lower capacities. Although NPC had significantly lower CO 2 capacity than SPC, its uptake performance could be improved by 21 wt% after H 2 reduction at 600 °C, producing reduced-NPC (R-NPC) with secondary amine groups ( Fig. 1a ). Even though the surface area of R-NPC (1,450 m 2 g −1 ) is only slightly greater than that of the activated carbon (1,430 m 2 g −1 ), the presence of the amine groups induces the formation of the poly(CO 2 ) under pressure, promoting the CO 2 sorption efficiency of the R-NPC. The pore volume of R-NPC is 1.43 cm 3 g −1 . 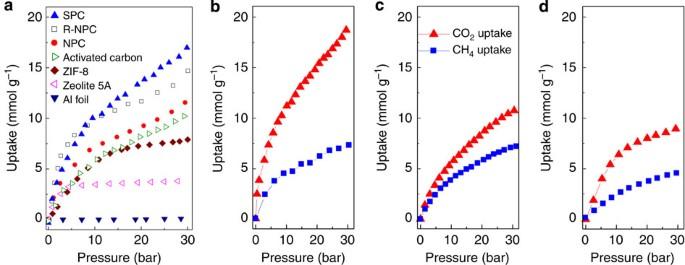Figure 4: Volumetric gas uptake data. (a) Volumetric CO2uptake performance at 30 °C of SPC, NPC, R-NPC and traditional sorbents: activated carbon, ZIF-8, and zeolite 5A. Al foil was used as a reference to ensure no CO2condensation was occurring in the system at this temperature and pressure. Volumetric CO2and CH4uptake tests at 23 °C on (b) SPC, (c) activated carbon and (d) ZIF-8 sorbents. Figure 4: Volumetric gas uptake data. ( a ) Volumetric CO 2 uptake performance at 30 °C of SPC, NPC, R-NPC and traditional sorbents: activated carbon, ZIF-8, and zeolite 5A. Al foil was used as a reference to ensure no CO 2 condensation was occurring in the system at this temperature and pressure. Volumetric CO 2 and CH 4 uptake tests at 23 °C on ( b ) SPC, ( c ) activated carbon and ( d ) ZIF-8 sorbents. Full size image Purification of natural gas from wells relies upon a highly CO 2 -selective sorbent, especially in a CH 4 -rich environment. Thus, CH 4 uptake experiments were carried out on three different types of porous materials, SPC, activated carbon and ZIF-8. Figure 4b–d compares CO 2 and CH 4 sorption over a pressure range from 0 to 30 bar at 23 °C. In contrast to the CO 2 sorption, the CH 4 isotherms for these three sorbents reached equilibrium while the system pressure was approaching 30 bar. The order of the CH 4 uptake capacities was correlated to the surface area of the sorbents. Comparing these sorbents, the observed molecular ratio of sorbed CO 2 to CH 4 ( n CO2 / n CH4 ) for the SPC (2.6) was greater than that for the activated carbon (1.5) and ZIF-8 (1.9). In addition, the density of the SPC calculated using volumetric analysis is sixfold higher than in the ZIF-8 (2.21 versus 0.35 g cm −3 ) and threefold higher than the zeolite 5A (2.21 versus 0.67 g cm −3 ). The high CO 2 capacity and high density observed for SPC greatly increase the volume efficiency, which would reduce the volume of the sorption material for a given CO 2 uptake production rate. In order to mimic a gas well environment and further characterize the SPC’s selectivity to CO 2 , a premixed gas (85 mol% CH 4 , 10 mol% CO 2 , 3 mol% C 2 H 6 and 2 mol% C 3 H 8 ) was used with quadrupole mass spectrometry (MS) detection. The MS inlet was connected to the gas uptake system so that it could monitor the gas effluent from the SPC throughout the sorption–desorption experiment. Supplementary Fig. 6 shows the mass spectrum recorded during the sorption process. The peaks at 15 and 16 amu correspond to fragment and molecular ions from CH 4 , while the peaks at 28 and 44 amu are from CO 2 in the premixed gas. Other minor peaks can be assigned to fragment ions from C 2 H 6 and C 3 H 8 . Although the peak at 44 amu can also come from C 3 H 8 ions, the contribution is negligible because of the lower C 3 H 8 concentration in the mixed gas, and it is distinguishable by the fragmentation ratios in the MS (C 3 H 8 : m / z =29 (100), 44 (30); CO 2 : m / z =44(100), 28(11)). The observed intensity ratio of two peaks at 16 and 44 amu ( I 16 / I 44 =9.1) indicates the abundance of CH 4 versus CO 2 during the sorption and also reflects the relative amount of CH 4 and CO 2 in the premixed gas. Once the sorption reached equilibrium under 30 bar, the desorption process was induced by slowly venting into the MS system. The I 16 / I 44 ratio reduced to ~0.7. The SPC has been shown to have 2.6-fold higher CO 2 than CH 4 affinity at 30 bar when using pure CO 2 and CH 4 as feed gases ( Fig. 4b ). If the binding energy of CH 4 and CO 2 were assumed to be similar, and the partial pressure of CH 4 versus CO 2 in the premixed gas is considered ( P CH4 / P CO2 =8.5), then the number of sorbed CH 4 should be ~3.3-times more than that of the sorbed CO 2 . Typically, CO 2 -selective materials have selective sites and once the CO 2 occupies those sites, the selectivity significantly decreases and the materials behave as a physisorbent with lower selectivities at higher pressures. On the contrary, here the SPC demonstrates much higher CO 2 selectivity than expected since the chemisorbed sulphur-initiated poly(CO 2 ) chain displaces physisorbed gas. Under the mechanism described here for CO 2 polymerization in the channels of inexpensive nucleophilic porous carbons, these new materials have continuous selectivity toward CO 2 , limited only by the available pore space and pressure. Through development of these enhanced stationary phase sorbents, capture and reinjection of CO 2 at the natural gas sites could be realized, thereby leading to greatly reduced CO 2 emissions from natural gas streams. CO 2 fixation through polymerization is disclosed here as a major advance for future capture and possibly storage of this greenhouse gas. Instrumentation at Rice University An automated Sieverts instrument (Setaram PCTPro) was adopted to measure gas (CO 2 , CH 4 or premixed gas) sorption properties of materials. Typically, ~70 mg of sorbent was packed into a ~1.3 ml of stainless steel sample cell. The sample was pretreated under vacuum (~3 mm Hg) at 130 °C for 6 h and the sample volume was further determined by helium before the uptake experiment. At each step of the measurement, testing gas was expanded from the reference reservoir into the sample cell until the system pressure reached equilibrium. A quadrupole mass spectrometer (Setaram RGA200) was connected to the Sieverts instrument so that it could monitor the gas effluent from the sorbent throughout the entire sorption–desorption experiment. With the assistance of a hybrid turbomolecular drag pump, the background pressure of the MS can be controlled lower than 5 × 10 −8 Torr. All material densities were determined using volumetric analysis on this same instrument. XPS was performed using a PHI Quantera SXM Scanning X-ray Microprobe with a base pressure of 5 × 10 −9 Torr. Survey spectra were recorded in 0.5 eV step size and a pass energy of 140 eV. Elemental spectra were recorded in 0.1 eV step size and a pass energy of 26 eV. All spectra were standardized using C1s peak (284.5 eV) as a reference. The ATR-IR experiment was conducted using a Fourier transform infrared spectrometer (Nicolet Nexus 670) equipped with an attenuated total reflectance system (Nicolet, Smart Golden Gate) and a MCT-A detector. Raman spectra were measured using a Renishaw inVia Raman Microscope with a 514 nm excitation argon laser. Scanning electron microscope images were taken at 15 KeV using a JEOL-6500 F field emission microscope. High-resolution TEM images were obtained with a JEOL 2100 F field emission gun TEM. An automated BET surface analyser (Quantachrome Autosorb-3b) was used for measurements of sorbents’ surface areas and pore volumes based on N 2 adsorption–desorption. Typically, a ~100 mg of sample was loaded into a quartz tube and pretreated at 130 °C under vacuum (~5 mm Hg) in order to remove sorbates before the measurement. MAS NMR spectra were recorded on a Bruker Avance III 4.7 T spectrometer with a standard MAS probe for 4 mm outer diameter rotors. Instrumentation at NIST Volumetric CO 2 sorption measurements were carried out on computer-controlled custom-built volumetric sorption equipment previously described in detail [23] , with an estimated reproducibility within 0.5% and isotherm data error bar of less than 2% compared with other commercial instruments. An amount of ~79 mg of sample was used for the experiments. Sample degassing, before the CO 2 sorption experiment, was done at 130 °C under vacuum for 12 h. Gravimetric CO 2 sorption measurements were performed on a high pressure thermal gravimetric equipment (Model: TGA-HP50) from TA Instruments. An amount of ~15 mg of sample was used for the experiments. Sample degassing, before CO 2 sorption experiment, was done at 130 °C under vacuum for 12 h. Synthesis of SPC Poly[(2-hydroxymethyl)thiophene] (PTh) (Sigma-Aldrich) was prepared using FeCl 3 (ref. 24 ) In a typical synthesis, 2-thiophenemethanol (1.5 g, 13.1 mmol) in CH 3 CN (10 ml) was slowly added under vigorous stirring to a slurry of FeCl 3 (14.5 g, 89.4 mmol) in CH 3 CN (50 ml). The mixture was stirred at room temperature for 24 h. The polymer (PTh) was separated by filtration over a sintered glass funnel, washed with distilled water (~1 l) and then with acetone (~200 ml). The polymer was dried at 100 °C for 12 h to afford 1.21 g (96% yield) of the desired compound. The PTh was activated by grinding PTh (500 mg) with KOH (1 g, 17.8 mmol) with a mortar and pestle and then heated under Ar at 600 °C in a tube furnace for 1 h. The Ar flow rate was 500 sccm. After cooling, the activated sample was thoroughly washed 3 × with 1.2 M HCl (1 l) and then with distilled water until the filtrate attained pH 7. The SPC sample was dried in an oven at 100 °C to afford 240 mg of the black solid SPC. The BET surface area and pore volume were 2,500 m 2 g −1 and 1.01 cm 3 g −1 , respectively. Synthesis of NPC Commercial polyacrylonitrile (PAN, 500 mg, average M w 150,000, Sigma-Aldrich) powder and KOH (1,500 mg, 26.8 mmol) were ground to a homogeneous mixture in a mortar. The mixture was subsequently carbonized by heating to 600 °C under Ar (500 sccm) in a tube furnace for 1 h. The carbonized material was washed 3 × with 1.2 M HCl (1 l) and then with distilled water until the filtrate attained pH 7. Finally, the carbon sample was dried in an oven at 100 °C to afford 340 mg of the solid black NPC. To produce R-NPC, the activated material (270 mg) was further reduced by 10% H 2 (H 2 :Ar=50:450 sccm) at 600 °C for 1 h to provide 255 mg of the final material. The BET surface area and pore volume were 1,450 m 2 g −1 and 1.43 cm 3 g −1 , respectively. How to cite this article : Hwang, C.-C. et al. Capturing carbon dioxide as a polymer from natural gas. Nat. Commun. 5:3961 doi: 10.1038/ncomms4961 (2014).